Modulation of β-catenin function maintains mouse epiblast stem cell and human embryonic stem cell self-renewal Wnt/β-catenin signalling has a variety of roles in regulating stem cell fates. Its specific role in mouse epiblast stem cell self-renewal, however, remains poorly understood. Here we show that Wnt/β-catenin functions in both self-renewal and differentiation in mouse epiblast stem cells. Stabilization and nuclear translocation of β-catenin and its subsequent binding to T-cell factors induces differentiation. Conversely, retention of stabilized β-catenin in the cytoplasm maintains self-renewal. Cytoplasmic retention of β-catenin is effected by stabilization of Axin2, a downstream target of β-catenin, or by genetic modifications to β-catenin that prevent its nuclear translocation. We also find that human embryonic stem cell and mouse epiblast stem cell fates are regulated by β-catenin through similar mechanisms. Our results elucidate a new role for β-catenin in stem cell self-renewal that is independent of its transcriptional activity and will have broad implications in understanding the molecular regulation of stem cell fate. Mouse epiblast stem cells (EpiSCs) are pluripotent stem cells derived from post-implantation epiblasts, and require the cytokines fibroblast growth factor 2 (FGF2) and activin A for self-renewal [1] , [2] . Mouse EpiSCs cultured in FGF2/activin survive poorly upon single-cell dissociation, and therefore are routinely passaged as small clumps. The lower viability of dissociated EpiSCs suggests that signalling pathways other than FGF2/activin might be involved in regulating EpiSC self-renewal. Although inhibition of Rho-associated kinase has been shown to protect cells from the apoptotic effects of single-cell dissociation [3] , it has no obvious effect in promoting self-renewal. We focused on Wnt/β-catenin as a candidate pathway for supporting EpiSC expansion, as it has been shown to have a central and conserved role in controlling cell proliferation and lineage specification during early embryogenesis [4] , [5] , and has also been implicated in promoting self-renewal of various types of stem cells [6] , [7] , [8] , [9] , [10] . In the absence of Wnt ligand, β-catenin, the key mediator of the canonical Wnt/β-catenin pathway, is phosphorylated by glycogen synthase kinase 3 (GSK3), leading to proteasome-mediated degradation of β-catenin. When Wnt ligand binds to its receptor complex, composed of frizzled and low-density-lipoprotein-receptor-related protein 5 or 6, the canonical Wnt/β-catenin pathway is activated, leading to the inhibition of GSK3 and the stabilization of β-catenin. Stabilized β-catenin then translocates to the nucleus, where it interacts with T-cell factors (TCFs) to regulate gene expression. Activation of Wnt/β-catenin signalling produces diverse and sometimes opposite outcomes in different cell types, and it has therefore been proposed that Wnt/β-catenin might regulate cell fates in a context- and cell type-dependent manner [11] . How activation of the same Wnt/β-catenin signal yields disparate effects in different cell types, however, remains poorly understood. Here we reveal a mechanism by which Wnt/β-catenin regulates stem cell fates. Wnt/β-catenin signalling promotes mouse EpiSC self-renewal when stabilized β-catenin is retained in the cytoplasm, and induces differentiation if β-catenin translocates into the nucleus and binds TCFs. Wnt/β-catenin also regulates human ESC fate through a mechanism similar to that in mouse EpiSCs. This supports the notion that human ESCs are more closely related to mouse EpiSCs than to mouse ESCs, which in a β-catenin-mediated self-renewal context are able to maintain self-renewal only when β-catenin binds TCFs [9] , [12] . Small molecules maintains EpiSC self-renewal Previously, we showed that two small-molecule inhibitors (2i), CHIR99021 (CHIR) and PD0325901, could efficiently maintain mouse ESC self-renewal independent of LIF/STAT3 signalling [9] . CHIR stabilizes β-catenin through inhibition of GSK3, and PD0325901 suppresses the mitogen-activated protein kinase pathway. To ascertain whether this inhibitor-based system is also capable of maintaining self-renewal in EpiSCs, we administered CHIR with or without PD0325901 and found that EpiSCs rapidly differentiated or died in both cases ( Supplementary Fig. S1a ). We therefore reasoned that if CHIR induces EpiSC differentiation through stabilization of β-catenin, de-stabilization of β-catenin might promote EpiSC self-renewal. We tested this hypothesis by administering the tankyrase inhibitor XAV939 to mouse EpiSC cultures. XAV939-mediated inhibition of tankyrase stabilizes Axin, leading to the formation of the β-catenin destruction complex, composed of GSK3, Axin and adenomatous polyposis coli (APC) [13] . In the presence of XAV939, mouse EpiSCs remained undifferentiated for ~1 week, but differentiated after passaging ( Supplementary Fig. S1b ). Surprisingly, dual administration of CHIR and XAV939 (‘CHIR/XAV’ hereafter) allowed long-term maintenance of undifferentiated EpiSCs without exogenous growth factors or cytokines ( Fig. 1a ). EpiSCs cultured in CHIR/XAV could be routinely passaged by single-cell dissociation and replating onto gelatin-coated dishes, and could be cryo-preserved and recovered at high efficiency by standard techniques. 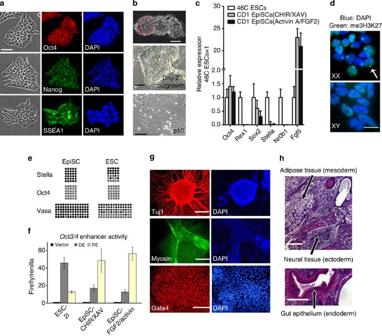Figure 1: Mouse EpiSCs maintained in CHIR and XAV retain pluripotency. (a) CD1 mouse EpiSCs were cultured in CHIR/XAV for seven passages and were subsequently immunostained with indicated antibodies against pluripotency markers. (b)De novoderivation of mouse EpiSCs. Epiblast tissue (outlined in red dashed line) of the E5.75 CD1 mouse embryo was dissected and cultured in CHIR/XAV. The outgrowth formed from the plated epiblast (middle panel) was disaggregated to establish a stable EpiSC line (right panel). Thirteen EpiSC lines were established from 13-plated CD1 mouse embryos. (c) qRT–PCR analysis of gene expression in mouse EpiSCs maintained in CHIR/XAV or FGF2/activin. Expression levels are relative to those of mouse ESCs maintained in 2i. Data represent mean±s.d. of triplicate samples from three independent experiments. (d) Immunostaining of male and female CD1 EpiSCs for me3H3K27. The nuclear focus indicated by the arrow is a mark of X chromosome inactivation. DAPI is a nuclear stain. (e) Bisulfite sequencing of DNA methylation of the promoter regions ofStella,Oct4andVasain mouse ESCs maintained in 2i and EpiSCs maintained in CHIR/XAV. (f) Quantification ofOct4distal enhancer (DE) and proximal enhancer (PE) reporter activities in mouse ESCs and EpiSCs. Data represent mean±s.d. of three experimental replicates. (g) Immunostaining showing Tuj- positive neurons (ectoderm), myosin-positive beating cardiomyocytes (mesoderm) and Gata4-positive endoderm cells derived from CD1 mouse EpiSCs through EBs formation. (h) Hematoxylin and eosin (H&E) staining of teratomas generated from CD1 mouse EpiSCs derived and cultured in CHIR/XAV. Upper, middle and bottom arrows indicate adipose tissue, neural tissue and gut epithelium, respectively. Scale bar, 50 μm (for panelsa,b,g,h); scale bar, 10 μm (for paneld). Figure 1: Mouse EpiSCs maintained in CHIR and XAV retain pluripotency. ( a ) CD1 mouse EpiSCs were cultured in CHIR/XAV for seven passages and were subsequently immunostained with indicated antibodies against pluripotency markers. ( b ) De novo derivation of mouse EpiSCs. Epiblast tissue (outlined in red dashed line) of the E5.75 CD1 mouse embryo was dissected and cultured in CHIR/XAV. The outgrowth formed from the plated epiblast (middle panel) was disaggregated to establish a stable EpiSC line (right panel). Thirteen EpiSC lines were established from 13-plated CD1 mouse embryos. ( c ) qRT–PCR analysis of gene expression in mouse EpiSCs maintained in CHIR/XAV or FGF2/activin. Expression levels are relative to those of mouse ESCs maintained in 2i. Data represent mean±s.d. of triplicate samples from three independent experiments. ( d ) Immunostaining of male and female CD1 EpiSCs for me3H3K27. The nuclear focus indicated by the arrow is a mark of X chromosome inactivation. DAPI is a nuclear stain. ( e ) Bisulfite sequencing of DNA methylation of the promoter regions of Stella , Oct4 and Vasa in mouse ESCs maintained in 2i and EpiSCs maintained in CHIR/XAV. ( f ) Quantification of Oct4 distal enhancer (DE) and proximal enhancer (PE) reporter activities in mouse ESCs and EpiSCs. Data represent mean±s.d. of three experimental replicates. ( g ) Immunostaining showing Tuj- positive neurons (ectoderm), myosin-positive beating cardiomyocytes (mesoderm) and Gata4-positive endoderm cells derived from CD1 mouse EpiSCs through EBs formation. ( h ) Hematoxylin and eosin (H&E) staining of teratomas generated from CD1 mouse EpiSCs derived and cultured in CHIR/XAV. Upper, middle and bottom arrows indicate adipose tissue, neural tissue and gut epithelium, respectively. Scale bar, 50 μm (for panels a , b , g , h ); scale bar, 10 μm (for panel d ). Full size image We compared the clonogenicity of EpiSCs cultured in different conditions. Approximately 13% of individual EpiSCs plated onto gelatin-coated 96-well plates and cultured in CHIR/XAV formed morphologically undifferentiated colonies. This colony formation frequency is approximately six times greater than that of EpiSCs cultured in FGF2/activin ( Supplementary Fig. S1c,d ). EpiSC colonies that formed in CHIR/XAV were readily expanded to establish stable cell lines. The high propagation efficiency in CHIR/XAV prompted us to test the derivation of EpiSC lines de novo in this condition. As expected, in the presence of CHIR/XAV, EpiSCs were readily derived from embryonic day (E) 5.75 embryos of CD1 and 129SvE mice ( Fig. 1b and Supplementary Fig. S1e ). EpiSCs were also established from E7.5 Sprague–Dawley and Dark Agouti rat embryos using CHIR/XAV ( Supplementary Fig. S1f,g ). To determine whether the cells derived and maintained in the CHIR/XAV condition retain an EpiSC identity, we examined their molecular and epigenetic profile and tested their differentiation potential. These cells expressed Oct4 and Sox2 , the key pluripotency genes, and Fgf5 , a post-implantation epiblast-specific marker [1] , [2] . Their expression of Rex1 , Nr0b1 and Stella , markers for the pre-implantation epiblast and primordial germ cells, was significantly lower than that of ESCs ( Fig. 1c ). Immunostaining for tri-methylated H3 lysine 27 (me3H3K27) on the X chromosome showed a large nuclear focus in each female EpiSC maintained in CHIR/XAV, indicating X chromosome silencing ( Fig. 1d ). In EpiSCs maintained in CHIR/XAV, the Oct4 promoter was unmethylated, while promoter regions of Stella and Vasa , specific markers for ESCs and primordial germ cells, were heavily methylated ( Fig. 1e ). EpiSCs maintained in CHIR/XAV showed strong activity in the Oct4 -proximal enhancer, which is preferentially active in EpiSCs, in contrast with ESCs, which mainly exhibit activity in the distal enhancer [14] , [15] ( Fig. 1f ). EpiSCs readily formed embryoid bodies (EBs) in suspension culture upon withdrawal of CHIR/XAV and differentiated into cell types representative of all three embryonic germ layers ( Fig. 1g ). We injected CD1 mouse EpiSCs derived and maintained in CHIR/XAV into two SCID mice. Teratomas containing tissues of all three embryonic germ layers were formed in both mice ( Fig. 1h ). We also tested the chimera formation ability of these CD1 EpiSCs by injecting them into C57BL/6 mouse blastocysts. No chimeras ensued from 58 blastocysts injected, an outcome consistent with previous observations [1] , [2] . To further establish the identity of EpiSCs maintained in CHIR/XAV, we performed whole-genome microarray analyses. EpiSCs derived and grown in CHIR/XAV or FGF2/activin exhibited similar gene expression patterns; these patterns were distinct from those of mouse ESCs ( Supplementary Fig. S2a ). Notably, expression of some ESC-specific genes, including Dppa2 , Dppa4 and Dppa5a [16] , [17] , was upregulated, whereas expression of the differentiation-associated genes Eomes and Nodal was downregulated in EpiSCs maintained in CHIR/XAV compared with EpiSCs in FGF2/activin ( Supplementary Fig. S2b ). These results suggest that although EpiSCs in CHIR/XAV exhibit key EpiSC features, they might be developmentally closer to ESCs than to EpiSCs grown in FGF2/activin. EpiSC self-renewal in CHIR/XAV is mediated by Axin2 Next, we investigated the mechanism by which CHIR/XAV promotes EpiSC self-renewal. By inhibiting GSK3 phosphorylation of β-catenin, CHIR stabilizes β-catenin, which then translocates to the nucleus and forms complexes with DNA-binding proteins, including TCFs, to activate transcription [5] . As expected, CHIR strongly induced β-catenin/TCF-responsive TOPFlash reporter activity in mouse EpiSCs; the addition of XAV significantly inhibited the TOPFlash activity induced by CHIR ( Fig. 2a ). We tested another small molecule, IWR-1, which, like XAV, also inhibits Wnt/β-catenin signalling through stabilization of Axin [18] . IWR-1 blocked TOPFlash reporter activity induced by CHIR, and the simultaneous presence of these inhibitors promoted EpiSC self-renewal. In contrast, IWP-2 and Pyrvinium, two small molecules that inhibit Wnt/β-catenin signalling through Axin stabilization-independent mechanisms [18] , [19] , were unable to support EpiSC self-renewal ( Fig. 2a,b ). These results prompted us to examine whether stabilization of Axin is necessary for EpiSC self-renewal promoted by XAV or IWR-1. There are two Axin genes, Axin1 and Axin2 . As expected, XAV or IWR-1 treatment significantly increased the amounts of both Axin1 and Axin2 in mouse EpiSCs ( Fig. 2c ). The expression level of Axin2, but not Axin1, was also elevated by CHIR treatment ( Fig. 2c ), an outcome consistent with previous findings that Axin2 is a direct downstream target of Wnt/β-catenin signalling [20] . As expected, the use of CHIR with either XAV or IWR-1 further increased the quantity of Axin2 protein in EpiSCs ( Fig. 2c ). To determine whether Axin mediates EpiSC self-renewal in CHIR/XAV or CHIR/IWR-1, we designed short hairpin RNAs (shRNAs) to knockdown Axin1 and Axin2. Interestingly, knockdown of Axin2, but not Axin1, impaired the self-renewal-promoting effect of CHIR/IWR-1 ( Fig. 2d–f ). To further test the influence of Axin on self-renewal, we established mouse EpiSCs overexpressing Axin1 (Axin1-EpiSCs) or Axin2 (Axin2-EpiSCs) in the FGF2/activin condition ( Fig. 2g ). Addition of CHIR failed to induce TOPFlash activity in Axin2-EpiSCs ( Supplementary Fig. S3 ). CHIR alone was sufficient to support robust and long-term expansion of undifferentiated Axin2-EpiSCs following the removal of FGF2/activin. In contrast, Axin1-EpiSCs rapidly differentiated in the presence of CHIR after the removal of FGF2/activin ( Fig. 2h ). Taken together, these results suggest that Axin2 is the key mediator of EpiSC self-renewal promoted by CHIR/IWR-1 or CHIR/XAV. 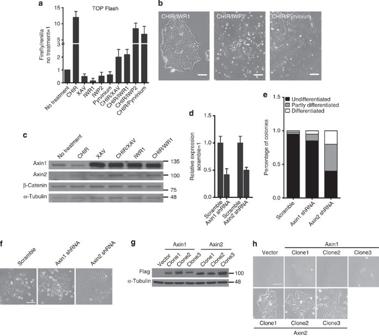Figure 2: Stabilization of Axin2 mediates self-renewal of EpiSCs maintained in CHIR and XAV or CHIR and IWR-1. (a) TOPFlash assay in CD1 mouse EpiSCs treated with the indicated inhibitors for 12 h. Data represent mean±s.d. of three biological replicates. (b) Representative phase contrast images of CD1 mouse EpiSCs cultured in the indicated conditions for 7 days. (c) Western blot analysis of CD1 mouse EpiSCs treated with the indicated inhibitors for 12 h. (d) qRT–PCR analysis ofAxin1andAxin2mRNA levels in CD1 mouse EpiSCs stably transfected with Axin1 shRNA or Axin2 shRNA. Data represent mean±s.d. of three biological replicates. (e) Colony assay on CD1 mouse EpiSCs stably transfected with scramble, Axin1 or Axin2 shRNAs. Cells were plated onto a six-well plate at a density of 5,000 cells per well and cultured in CHIR/IWR-1. Colonies were counted 7 days after plating. Data represent the total combined numbers of colonies from two independent experiments in which each shRNA-transfected group was cultured in one well of a six-well plate. (f) Representative phase contrast images of CD1 mouse EpiSCs stably transfected with the indicated shRNAs and cultured in CHIR/IWR-1 for 7 days. (g) Western blot analysis of CD1 mouse EpiSCs overexpressing Flag-tagged Axin1 or Axin2. (h) Representative phase contrast images of CD1 mouse EpiSCs overexpressing Axin1 or Axin2 and cultured in CHIR for 7 days. Axin2-overexpressing EpiSCs could be continually passaged in CHIR alone. Scale bar, 50 μm (for panelsb,f,h). Figure 2: Stabilization of Axin2 mediates self-renewal of EpiSCs maintained in CHIR and XAV or CHIR and IWR-1. ( a ) TOPFlash assay in CD1 mouse EpiSCs treated with the indicated inhibitors for 12 h. Data represent mean±s.d. of three biological replicates. ( b ) Representative phase contrast images of CD1 mouse EpiSCs cultured in the indicated conditions for 7 days. ( c ) Western blot analysis of CD1 mouse EpiSCs treated with the indicated inhibitors for 12 h. ( d ) qRT–PCR analysis of Axin1 and Axin2 mRNA levels in CD1 mouse EpiSCs stably transfected with Axin1 shRNA or Axin2 shRNA. Data represent mean±s.d. of three biological replicates. ( e ) Colony assay on CD1 mouse EpiSCs stably transfected with scramble, Axin1 or Axin2 shRNAs. Cells were plated onto a six-well plate at a density of 5,000 cells per well and cultured in CHIR/IWR-1. Colonies were counted 7 days after plating. Data represent the total combined numbers of colonies from two independent experiments in which each shRNA-transfected group was cultured in one well of a six-well plate. ( f ) Representative phase contrast images of CD1 mouse EpiSCs stably transfected with the indicated shRNAs and cultured in CHIR/IWR-1 for 7 days. ( g ) Western blot analysis of CD1 mouse EpiSCs overexpressing Flag-tagged Axin1 or Axin2. ( h ) Representative phase contrast images of CD1 mouse EpiSCs overexpressing Axin1 or Axin2 and cultured in CHIR for 7 days. Axin2-overexpressing EpiSCs could be continually passaged in CHIR alone. Scale bar, 50 μm (for panels b , f , h ). Full size image EpiSC self-renewal mediated by Axin2 is β-Catenin-dependent Next, we investigated how Axin2 mediates EpiSC self-renewal. We first sought to determine whether β-catenin is required for EpiSC self-renewal mediated by Axin2. We derived EpiSCs from mouse embryos carrying floxed alleles for β -catenin ( Fig. 3a,b ). Stable β -catenin −/− EpiSC lines were generated from these β -catenin fl/fl EpiSCs by transient transfection of Cre recombinase, and could be routinely maintained in FGF2/activin. Loss of β-catenin in these β -catenin −/− EpiSCs was confirmed by western blot analysis and the TOPFlash reporter assay ( Fig. 3c,d ). β -catenin −/− EpiSCs remained undifferentiated even after long-term culture in FGF2/activin, as suggested by EpiSC marker gene expression ( Fig. 3e,f ). However, they differentiated after the removal of FGF2/activin, even in the presence of CHIR/XAV or CHIR/IWR-1 ( Fig. 3g ), suggesting that EpiSC self-renewal in CHIR/XAV or CHIR/IWR-1 is likely mediated by β-catenin. To further confirm the role of β-catenin, we generated β -catenin −/− EpiSCs overexpressing Axin2 in the FGF2/activin condition ( Fig. 3h ). These cells differentiated after the removal of FGF2/activin, even in the presence of CHIR ( Fig. 3i ), suggesting that EpiSC self-renewal maintained by Axin2 is also β-catenin-dependent. 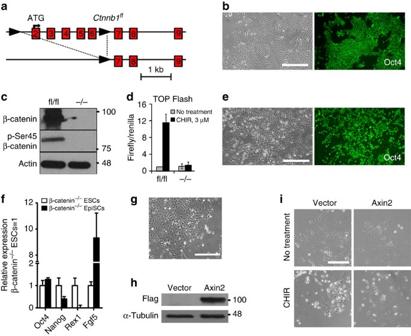Figure 3: Axin2-mediated EpiSC self-renewal is β-catenin-dependent. (a) Locus map of the mouse genome withloxP sites located in introns 1 and 6 of theCtnnb1(β-catenin) gene. Expression of Cre recombinase excises exons 2–6. (b) Immunocytochemistry showing strong Oct4 staining in most β-cateninfl/flEpiSCs derived and maintained in FGF2/activin. (c) Western blot analysis confirming the loss of β-catenin in β-catenin−/−EpiSCs. (d) TOPFlash assay in β-cateninfl/fland β-catenin−/−EpiSCs treated with 3 μM CHIR for 12 h. Data represent mean±s.d. of three biological replicates. (e) Immunocytochemistry showing strong Oct4 staining in most β-catenin−/−EpiSCs maintained in FGF2/activin. (f) qRT–PCR analysis of gene expression in β-catenin−/−ESCs and EpiSCs. Data represent mean±s.d. of three biological replicates. (g) Representative image of β-catenin−/−EpiSCs cultured in CHIR/XAV for 7 days after the removal of FGF2/activin. In the absence of FGF2/activin, β-catenin−/−EpiSCs cultured in basal medium (GMEM/10% FBS) or basal medium supplemented with CHIR/XAV or CHIR/IWR-1 differentiated and could not be maintained beyond passage 2 or 3. (h) Western blot analysis of β-catenin−/−EpiSCs overexpressing Flag-tagged Axin2. β-catenin−/−EpiSCs transfected with an empty vector were used as a control. (i) Representative phase contrast image of β-catenin−/−EpiSCs overexpressing Flag-tagged Axin2 and cultured in basal medium only (no treatment) or basal medium plus 3 μM CHIR for 7 days after the removal of FGF2/activin. Scale bar, 50 μm (for panelsb,e,g,i). Figure 3: Axin2-mediated EpiSC self-renewal is β-catenin-dependent. ( a ) Locus map of the mouse genome with lox P sites located in introns 1 and 6 of the Ctnnb1 (β -catenin ) gene. Expression of Cre recombinase excises exons 2–6. ( b ) Immunocytochemistry showing strong Oct4 staining in most β -catenin fl/fl EpiSCs derived and maintained in FGF2/activin. ( c ) Western blot analysis confirming the loss of β-catenin in β -catenin −/− EpiSCs. ( d ) TOPFlash assay in β -catenin fl/fl and β -catenin −/− EpiSCs treated with 3 μM CHIR for 12 h. Data represent mean±s.d. of three biological replicates. ( e ) Immunocytochemistry showing strong Oct4 staining in most β -catenin −/− EpiSCs maintained in FGF2/activin. ( f ) qRT–PCR analysis of gene expression in β -catenin −/− ESCs and EpiSCs. Data represent mean±s.d. of three biological replicates. ( g ) Representative image of β -catenin −/− EpiSCs cultured in CHIR/XAV for 7 days after the removal of FGF2/activin. In the absence of FGF2/activin, β -catenin −/− EpiSCs cultured in basal medium (GMEM/10% FBS) or basal medium supplemented with CHIR/XAV or CHIR/IWR-1 differentiated and could not be maintained beyond passage 2 or 3. ( h ) Western blot analysis of β -catenin −/− EpiSCs overexpressing Flag-tagged Axin2. β -catenin −/− EpiSCs transfected with an empty vector were used as a control. ( i ) Representative phase contrast image of β -catenin −/− EpiSCs overexpressing Flag-tagged Axin2 and cultured in basal medium only (no treatment) or basal medium plus 3 μM CHIR for 7 days after the removal of FGF2/activin. Scale bar, 50 μm (for panels b , e , g,i ). Full size image Cytoplasmic β-catenin mediates EpiSC self-renewal Next, we investigated how β-catenin mediates EpiSC self-renewal. Nuclear translocation of β-catenin and its subsequent binding to TCFs have been considered essential events in canonical Wnt/β-catenin signalling. To determine whether nuclear translocation of β-catenin is affected by Axin, we analysed β-catenin protein levels in whole-cell, cytoplasmic and nuclear fractions before and after CHIR treatment. The amounts of total and cytoplasmic β-catenin protein in Axin2-EpiSCs were comparable to those in EpiSCs transfected with vector only (vector-EpiSCs) ( Fig. 4a ); however, nuclear β-catenin in Axin2-EpiSCs was barely detectable before or after CHIR treatment, while CHIR treatment dramatically increased the nuclear β-catenin protein level in vector-EpiSCs and Axin1-EpiSCs ( Fig. 4a ). These results suggest that Axin2 overexpression does not lead to β-catenin degradation, but instead blocks nuclear translocation of β-catenin induced by CHIR. In Axin2-EpiSCs, Axin2 expression was mainly detected in the cytoplasm ( Fig. 4a,b ). Axin2 and β-catenin associated with each other, as shown by co-immunoprecipitation (Co-IP) ( Fig. 4c ); however, a physical association between β-catenin and TCF3 was barely detectable in Axin2-EpiSCs, even in the presence of CHIR ( Fig. 4c ). Taken together, these results suggest that Axin2 binds β-catenin and retains it in the cytoplasm, preventing its nuclear translocation and binding to TCFs. 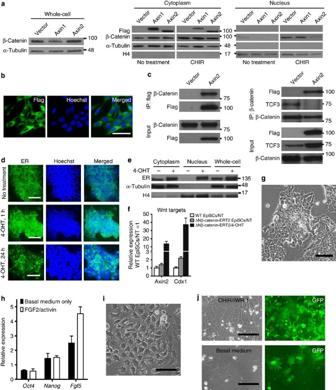Figure 4: Retention of stabilized β-catenin in the cytoplasm maintains EpiSC self-renewal. (a) Western blot analysis of cytoplasmic, nuclear and total β-catenin levels in CD1 mouse EpiSCs overexpressing Flag-tagged Axin1 or Axin2. Cells were either untreated or treated with 3 μM CHIR for 12 h. (b) Immunostaining of CD1 mouse EpiSCs overexpressing Flag-tagged Axin2. (c) Co-IP of Flag or β-catenin in CD1 mouse EpiSCs overexpressing empty vector or Flag-tagged Axin2. Cells were treated with 3 μM CHIR for 12 h. (d) Immunostaining of ΔNβ-catenin-ERT2-overexpressing CD1 mouse EpiSCs before and after treatment with 1 μM 4-OHT. (e) Western blot analysis of cytoplasmic and nuclear ΔNβ-catenin-ERT2 levels after treatment with 1 μM 4-OHT for 24 h. (f) qRT–PCR analysis ofAxin2andCdx1expression in wild-type and ΔNβ-catenin-ERT2 EpiSCs in basal medium or in the presence of 4-OHT for 12 h. Data represent mean±s.d. of three biological replicates. (g) A representative phase contrast image of ΔNβ-catenin-ERT2 EpiSCs after 25 passages in basal medium only. (h) qRT–PCR analysis ofOct4,NanogandFgf5mRNA levels in ΔNβ-catenin-ERT2-EpiSCs maintained in basal medium or basal medium plus FGF2/activin for 11 passages. Data represent mean±s.d. of three biological replicates. (i) Phase contrast image of ΔNβ-catenin-ERT2-EpiSCs after treatment with 1 μM 4-OHT for 24 h. (j) Phase contrast and fluorescent images of floxed ΔNβ-catenin-ERT2-EpiSCs cultured in the indicated conditions for 7 days after Cre-recombinase-mediated excision of the ΔNβ-catenin-ERT2 transgene. GFP expression was driven by the constitutive CAG promoter after excision of the floxed ΔNβ-catenin-ERT2-STOP cassette. Scale bar, 50 μm (for panelsb,d,g,i,j). Figure 4: Retention of stabilized β-catenin in the cytoplasm maintains EpiSC self-renewal. ( a ) Western blot analysis of cytoplasmic, nuclear and total β-catenin levels in CD1 mouse EpiSCs overexpressing Flag-tagged Axin1 or Axin2. Cells were either untreated or treated with 3 μM CHIR for 12 h. ( b ) Immunostaining of CD1 mouse EpiSCs overexpressing Flag-tagged Axin2. ( c ) Co-IP of Flag or β-catenin in CD1 mouse EpiSCs overexpressing empty vector or Flag-tagged Axin2. Cells were treated with 3 μM CHIR for 12 h. ( d ) Immunostaining of ΔNβ-catenin-ERT2-overexpressing CD1 mouse EpiSCs before and after treatment with 1 μM 4-OHT. ( e ) Western blot analysis of cytoplasmic and nuclear ΔNβ-catenin-ERT2 levels after treatment with 1 μM 4-OHT for 24 h. ( f ) qRT–PCR analysis of Axin2 and Cdx1 expression in wild-type and ΔNβ-catenin-ERT2 EpiSCs in basal medium or in the presence of 4-OHT for 12 h. Data represent mean±s.d. of three biological replicates. ( g ) A representative phase contrast image of ΔNβ-catenin-ERT2 EpiSCs after 25 passages in basal medium only. ( h ) qRT–PCR analysis of Oct4 , Nanog and Fgf5 mRNA levels in ΔNβ-catenin-ERT2-EpiSCs maintained in basal medium or basal medium plus FGF2/activin for 11 passages. Data represent mean±s.d. of three biological replicates. ( i ) Phase contrast image of ΔNβ-catenin-ERT2-EpiSCs after treatment with 1 μM 4-OHT for 24 h. ( j ) Phase contrast and fluorescent images of floxed ΔNβ-catenin-ERT2-EpiSCs cultured in the indicated conditions for 7 days after Cre-recombinase-mediated excision of the ΔNβ-catenin-ERT2 transgene. GFP expression was driven by the constitutive CAG promoter after excision of the floxed ΔNβ-catenin-ERT2-STOP cassette. Scale bar, 50 μm (for panels b , d , g , i , j ). Full size image To determine whether retention of β-catenin in the cytoplasm is necessary and sufficient for EpiSC self-renewal mediated by Axin2, we introduced a floxed ΔNβ-catenin-ERT2 (estrogen ligand-binding domain) transgene into mouse EpiSCs. ΔNβ-catenin-ERT2 is a fusion protein containing an N-terminally truncated, stabilized β-catenin and a mutant ERT2 (ref. 21 ). In the absence of 4-hydroxytamoxifen (4-OHT), ΔNβ-catenin-ERT2 remains in the cytoplasm. Administration of 4-OHT results in the translocation of ΔNβ-catenin-ERT2 into the nucleus, as confirmed by immunocytochemistry staining and immunoblotting ( Fig. 4d,e ), and activates the Wnt/β-catenin signalling pathway, as indicated by the increased expression of Wnt/β-catenin targets Axin2 and Cdx1 ( Fig. 4f ). EpiSCs overexpressing ΔNβ-catenin-ERT2 were expanded continuously for more than 25 passages in basal medium without addition of exogenous cytokines or small molecules, while retaining an EpiSC identity ( Fig. 4g,h ). The addition of 4-OHT resulted in rapid differentiation, even in the presence of IWR-1 ( Fig. 4i ). These results are likely attributable to the presence of the ΔNβ-catenin-ERT2 transgene, as its excision by Cre recombinase was associated with reversion to a wild-type EpiSC-like phenotype ( Fig. 4j ). Collectively, these results suggest that retention of stabilized β-catenin in the cytoplasm is necessary and sufficient for EpiSC self-renewal mediated by Axin2, and that nuclear β-catenin induces EpiSC differentiation. To further elaborate the role of β-catenin in EpiSCs, we generated a ΔNβ-catenin mutant containing two point mutations, at A295 and I296 (referred to as A295W/I296W hereafter). These point mutations render β-catenin unable to bind TCFs as well as Axin and APC [22] . β -catenin −/− EpiSCs overexpressing ΔNβ-catenin or ΔNβ-catenin/A295W/I296W were established in FGF2/activin. Although ΔNβ-catenin/A295W/I296W was present in the cytoplasm and nucleus of ΔNβ-catenin/A295W/I296W-expressing cells ( Supplementary Fig. S4a ), these cells exhibited no TOPFlash activity even in the presence of CHIR, whereas ΔNβ-catenin cells exhibited a high level of TOPFlash activity in the absence and presence of CHIR ( Supplementary Fig. S4b ). β -catenin −/− EpiSCs overexpressing ΔNβ-catenin rapidly differentiated after the removal of FGF2/activin. In contrast, β -catenin −/− EpiSCs overexpressing ΔNβ-catenin/A295W/I296W could be continuously expanded in basal medium without overt differentiation ( Supplementary Fig. S4c ). As nuclear β-catenin is mainly associated with TCFs, our results suggest that EpiSC differentiation induced by nuclear β-catenin is likely mediated by β-catenin–TCF binding; nonetheless, the interaction of β-catenin with Axin and APC conceivably might also contribute to the observed effects. A recent report has suggested that β-catenin forms a complex with Oct4 and E-cadherin in the membrane and this complex is involved in regulating ESC self-renewal and differentiation [23] . Next, we investigated whether membrane-bound β-catenin also has a role in the maintenance of EpiSCs. β-catenin is recruited to the cell membrane mainly through binding to E-cadherin [24] . We converted E-cadherin −/− mouse ESCs to EpiSCs under the FGF2/activin condition. These E-cadherin −/− EpiSCs could be expanded in CHIR/IWR-1, and retained an EpiSC identity ( Supplementary Fig. S4d,e ), indicating that membrane-bound β-catenin is likely not required for EpiSC self-renewal mediated by Axin2 and β-catenin. Modulating β-catenin function maintains human ESC self-renewal As human ESCs share defining features with mouse EpiSCs [2] , [25] , [26] , we tested whether modulating β-catenin function can also promote human ESC self-renewal. As was the case in mouse EpiSCs, TOPFlash reporter activity in human ESCs was strongly induced by CHIR; addition of either XAV or IWR-1 abolished this TOPFlash activity, while IWP-2 only partially suppressed such activity ( Fig. 5a ). Next, we examined the effect of CHIR/XAV and CHIR/IWR-1 on human ESC self-renewal. CHIR induced differentiation of human ESCs. In contrast, administration of CHIR with either XAV or IWR-1 resulted in robust self-renewal of human ESCs ( Fig. 5b ). We found that CHIR/IWR-1 is more effective than CHIR/XAV in promoting human ESC self-renewal, especially in feeder- and FGF2-free conditions; therefore, we focused on CHIR/IWR-1 for our human ESC study. Supplementation of conventional human ESC medium with CHIR/IWR-1 allowed robust propagation of Human ESCs; moreover, the clonogenicity of human ESCs cultured in CHIR/IWR-1 was significantly greater than that in the FGF2 condition ( Fig. 5c ). Human ESCs maintained in CHIR/IWR-1 express pluripotency markers Oct4, Nanog and Sox2 ( Fig. 5d ), and retain the ability to differentiate into cells of all three germ layers, both in vitro and in vivo ( Fig. 5e,f ). These results indicate that CHIR/IWR-1 mediates similar self-renewal responses in human ESCs and mouse EpiSCs. 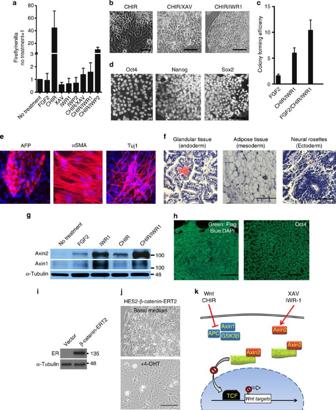Figure 5: β-catenin mediates human ESC self-renewal through a mechanism similar to that in mouse EpiSCs. (a) TOPFlash assay in H9 human ESCs subjected to the indicated treatments for 24 h. Data represent mean±s.d. of three biological replicates. (b) Representative phase contrast images of H9 human ESCs cultured in the indicated conditions for three passages (CHIR) or 11 passages (CHIR/XAV and CHIR/IWR-1). (c) Colony-forming efficiency assay of H9 human ESCs cultured in FGF2, CHIR/IWR-1 or FGF2/CHIR/IWR-1 conditions. Data represent mean±s.d. of three biological replicates. (d) H9 human ESCs cultured in CHIR/IWR-1 for 11 passages were immunostained with the indicated antibodies. (e) EBs were generated from H9 human ESCs cultured in CHIR/IWR-1 for 11 passages. The outgrowths of EBs were immunostained with the indicated antibodies. (f) H&E staining of teratomas generated from H9 ESCs cultured in CHIR/IWR-1 for 20 passages. (g) Western blot analysis of Axin1 and Axin2 expression in HES3 human ESCs treated with the indicated cytokines/inhibitors for 24 h. (h) Immunofluorescence images of H9 human ESCs (passage 5 in CHIR) overexpressing Flag-tagged Axin2. (i) Western blot analysis of ΔNβ-catenin-ERT2 expression in HES2 human ESCs with ER antibody. (j) Top panel: (a) representative phase contrast image of HES2 human ESCs overexpressing ΔNβ-catenin-ERT2 at passage six in basal medium only. These cells were cultured in basal medium only for more than 15 passages and remained morphologically undifferentiated. Bottom panel: 3 days after treatment with 1 μM 4-OHT, nearly all the HES2-ΔNβ-catenin-ERT2 human ESCs differentiated. (k) Model of mouse EpiSC and human ESC self-renewal mediated by β-catenin. In the absence of Wnt or GSK3 inhibitor, a β-catenin destruction complex, containing Axin1, GSK3 and APC is formed, leading to the degradation of β-catenin and differentiation. In the presence of Wnt or GSK3 inhibitor, β-catenin is stabilized and can initiate cellular responses related to both self-renewal and differentiation. Stabilized β-catenin induces differentiation when it translocates into the nucleus and binds TCFs to activate downstream targets. Addition of XAV or IWR-1 stabilizes Axin2. Stabilized Axin2 binds β-catenin and retains it in the cytoplasm, resulting in self-renewal through a yet unknown mechanism. Scale bar, 50 μm (for panelsb,d,e,f,h,j). Figure 5: β-catenin mediates human ESC self-renewal through a mechanism similar to that in mouse EpiSCs. ( a ) TOPFlash assay in H9 human ESCs subjected to the indicated treatments for 24 h. Data represent mean±s.d. of three biological replicates. ( b ) Representative phase contrast images of H9 human ESCs cultured in the indicated conditions for three passages (CHIR) or 11 passages (CHIR/XAV and CHIR/IWR-1). ( c ) Colony-forming efficiency assay of H9 human ESCs cultured in FGF2, CHIR/IWR-1 or FGF2/CHIR/IWR-1 conditions. Data represent mean±s.d. of three biological replicates. ( d ) H9 human ESCs cultured in CHIR/IWR-1 for 11 passages were immunostained with the indicated antibodies. ( e ) EBs were generated from H9 human ESCs cultured in CHIR/IWR-1 for 11 passages. The outgrowths of EBs were immunostained with the indicated antibodies. ( f ) H&E staining of teratomas generated from H9 ESCs cultured in CHIR/IWR-1 for 20 passages. ( g ) Western blot analysis of Axin1 and Axin2 expression in HES3 human ESCs treated with the indicated cytokines/inhibitors for 24 h. ( h ) Immunofluorescence images of H9 human ESCs (passage 5 in CHIR) overexpressing Flag-tagged Axin2. ( i ) Western blot analysis of ΔNβ-catenin-ERT2 expression in HES2 human ESCs with ER antibody. ( j ) Top panel: ( a ) representative phase contrast image of HES2 human ESCs overexpressing ΔNβ-catenin-ERT2 at passage six in basal medium only. These cells were cultured in basal medium only for more than 15 passages and remained morphologically undifferentiated. Bottom panel: 3 days after treatment with 1 μM 4-OHT, nearly all the HES2-ΔNβ-catenin-ERT2 human ESCs differentiated. ( k ) Model of mouse EpiSC and human ESC self-renewal mediated by β-catenin. In the absence of Wnt or GSK3 inhibitor, a β-catenin destruction complex, containing Axin1, GSK3 and APC is formed, leading to the degradation of β-catenin and differentiation. In the presence of Wnt or GSK3 inhibitor, β-catenin is stabilized and can initiate cellular responses related to both self-renewal and differentiation. Stabilized β-catenin induces differentiation when it translocates into the nucleus and binds TCFs to activate downstream targets. Addition of XAV or IWR-1 stabilizes Axin2. Stabilized Axin2 binds β-catenin and retains it in the cytoplasm, resulting in self-renewal through a yet unknown mechanism. Scale bar, 50 μm (for panels b , d , e , f , h , j ). Full size image Next, we investigated whether CHIR/IWR-1 maintains human ESC self-renewal through a mechanism similar to that in mouse EpiSCs. IWR-1 treatment significantly increased the amounts of both Axin1 and Axin2 in human ESCs. CHIR induced the expression of Axin2, but not Axin1, and combined use of CHIR with IWR-1 further increased Axin2 protein level ( Fig. 5g ), an outcome similar to what we observed in mouse EpiSCs. To confirm whether Axin2 also mediates human ESC self-renewal, we stably introduced an Axin2 transgene into human ESCs (Axin2-hESC). As expected, CHIR, administrated alone, could support stable and long-term self-renewal of Axin2-hESCs ( Fig. 5h ). Finally, to determine whether cytoplasmic β-catenin can also promotes human ESC self-renewal, we introduced the ΔNβ-catenin-ERT2 transgene into human ESCs ( Fig. 5i ). As expected, human ESCs overexpressing ΔNβ-catenin-ERT2 could be continually passaged without overt differentiation, whereas addition of 4-OHT induced rapid differentiation ( Fig. 5j ). These results suggest that human ESC self-renewal and mouse EpiSC self-renewal are supported by a similar mechanism: an increased level of cytoplasmic β-catenin and the prevention of β-catenin–TCF interaction. Our study demonstrates that Wnt/β-catenin signalling can promote self-renewal or differentiation of mouse EpiSCs and human ESCs. The retention of stabilized β-catenin in the cytoplasm maintains mouse EpiSC and human ESC self-renewal, whereas nuclear translocation of β-catenin and subsequent binding to TCFs induces differentiation ( Fig. 5k ). Our finding that cytoplasmic and nuclear β-catenin pools are both involved in regulating cell fates might provide a rational explanation for some of the diverse and sometimes opposite effects of Wnt/β-catenin observed in different contexts. More importantly, our study reveals a new functional avenue of the canonical Wnt/β-catenin pathway, which current dogma depicts as being functionally defined by nuclear translocation of β-catenin and its subsequent binding to TCFs. The gene regulatory effects of Wnt/β-catenin signalling are initiated upon the binding of β-catenin to TCFs in the nucleus. So how is cytoplasmic β-catenin involved in regulating cell fates? One possible model of regulation is suggested by the interaction of cytoplasmic β-catenin with cadherin, α-catenin and actin filaments [27] , as these interactions have been shown to have multiple and important roles in regulating cellular organization, cell adhesion and signal transduction from cell surface to the nucleus. Another possibility is that cytoplasmic β-catenin might hold negative regulators of self-renewal in the cytoplasm, preventing them from entering the nucleus and activating or suppressing transcription of their target genes. In this scenario, cytoplasmic β-catenin would promote stem cell self-renewal by alleviating the self-renewal suppression effect of these negative regulators. This might be the case in mouse EpiSCs and human ESCs in which the persistence of β-catenin in the cytoplasm is associated with self-renewal. The role of β-catenin in human ESC self-renewal has been controversial. It has been suggested that activation of β-catenin by Wnt ligands or GSK3 inhibitors can promote human ESC self-renewal [28] , [29] . Other studies showed that Wnt/β-catenin signalling is dispensable for human ESC self-renewal, and that its activation predominantly induces differentiation [30] , [31] . Our finding that activation of β-catenin can promote human ESC self-renewal or differentiation, and that the respective outcome is dictated by whether β-catenin translocates into the nucleus, provides a rational explanation for earlier, seemingly paradoxical results. We also found that FGF2 and CHIR/IWR-1 act synergistically to promote human ESC self-renewal ( Fig. 5c ). This is noteworthy because in mouse ESCs, LIF and CHIR/PD can also independently promote self-renewal, yet there is a synergistic effect when the two are combined [32] , [33] . Understanding how these different pathways work independently or synergistically to maintain stem cell self-renewal will advance our efforts to better control stem cell fate, which is critical to the future of regenerative medicine. Small-molecule inhibitors and cytokines The following small-molecule inhibitors and cytokines were used at the indicated final concentrations: CHIR99021 (3 μM), PD0325901 (1 μM), XAV939 (Sigma, 2 μM), IWR-1 (Sigma, 2.5 μM), IWP-2 (Stemgent, 2.5 μM), Pyrvinium (Sigma, 100 nM), recombinant human FGF2 (PeproTech, 10 ng ml −1 ), and recombinant human activin A (PeproTech, 10 ng ml −1 ). CHIR99021 and PD0325901 were synthesized in the Division of Signal Transduction Therapy, University of Dundee, UK. Culture media for mouse and rat EpiSCs, and human ESCs The basal medium for mouse EpiSC culture is the conventional mouse ESC medium, which consists of GMEM (Sigma) supplemented with 10% fetal bovine serum (FBS) (Hyclone), 2 mM L -glutamine (Invitrogen), 1 mM sodium pyruvate (Invitrogen), 1% non-essential amino acids (Invitrogen) and 0.1 mM β-mercaptoethanol. Mouse EpiSCs were derived and maintained in the basal medium supplemented with FGF2/activin, CHIR/XAV or CHIR/IWR-1. The basal medium for rat EpiSC culture is N2B27, which was prepared by mixing 500 ml of DMEM/F12 (Invitrogen) with 500 ml of neurobasal medium (Invitrogen) and adding 5 ml of N 2 (Invitrogen), 10 ml of B27 (Invitrogen), 5 ml of glutamax (Invitrogen), and 1 ml of 0.1 M β-mercaptoethanol (Sigma) [34] . The basal medium for human ESC culture consists of Knockout DMEM/F12 supplemented with 20% Knockout serum replacement (KSR) (Invitrogen), 1% non-essential amino acids, 2 mM L -glutamine and 0.1 mM β-mercaptoethanol. Human ESCs were cultured in the basal medium supplemented with FGF2, CHIR/XAV or CHIR/IWR-1. Derivation and propagation of EpiSCs Post-implantation epiblasts were isolated from E5.75 mouse embryos or E7.5 rat embryos and dissociated into small clumps with 0.05% trypsin [35] . Epiblast fragments were placed into four-well plates pre-coated with 0.1% gelatin (for mouse epiblasts) or pre-seeded with γ-irradiated mouse embryonic fibroblasts (MEFs) (for rat epiblasts) and cultured in either the FGF2/activin or the CHIR/XAV conditions. Emerging EpiSCs were trypsinized and expanded every 2–3 days at a subculture ratio of 1:4. Animal experiments were performed according to the investigator’s protocols approved by the University of Southern California Institutional Animal Care and Use Committee. Human ESC culture H1, H9, HES2 and HES3 human ESC lines were kindly provided by the University of Southern California Stem Cell Core Facility. Human ESCs were routinely maintained on γ-irradiated MEF feeders in human ESC basal medium supplemented with 10 ng ml −1 FGF2. For culture in the CHIR/IWR-1 or CHIR/XAV condition, human ESCs were plated onto dishes pre-coated with Matrigel (BD Biosciences) or pre-seeded with MEFs and cultured in the basal medium supplemented with 3 μM CHIR99021, 2.5 μM IWR-1 or 2 μM XAV939. For passaging, human ESCs were dissociated into single cells with 0.05% trypsin or small clumps with the Calcium Trypsin KSR(CTK) solution every 2–4 days [36] , and replated into the CHIR/IWR-1 or CHIR/XAV condition. To evaluate the colony-forming efficiency of human ESCs cultured in FGF2, CHIR/IWR-1 or FGF2/CHIR/IWR-1 condition, cells were trypsinized and passed through 40 μm cell strainer (BD Biosciences) to obtain single-cell suspension. Cells were then counted and seeded at a density of 1,000 cells per well onto six-well plates pre-seeded with MEFs. After 7 days, cells were fixed with 4% paraformaldehyde and stained for alkaline phosphatase (AP) using the Vector Blue Substrate kit (Vector laboratories). Colony-forming efficiencies were calculated as the number of AP-positive colonies formed divided by the number of cells plated. Generation of β -catenin −/− mouse EpiSCs and ESCs β -catenin fl/fl EpiSCs were derived from B6.129- Ctnnb1 tm2Kem /KnwJ mice (The Jackson Laboratory) that possess lox P sites located in introns 1 and 6 of the Ctnnb1 (β -catenin ) gene [37] . β -catenin fl/fl EpiSCs were derived and maintained in the FGF2/activin condition. β -catenin −/− ESCs were generated from β -catenin fl/fl ESCs by transient transfection of the pCAG-Cre-IRES-Puro plasmid using Lipofectamine (Invitrogen). Transfectants were selected for 7 days in GMEM/10% FBS medium supplemented with 10 ng ml −1 LIF, 1 μM PD0325901 and 1 μg ml −1 puromycin. Puromycin-resistant ESC colonies were picked and expanded in the LIF+PD0325901 condition (LIF alone was not sufficient to maintain self-renewal of β -catenin −/− ESCs). Loss of β-catenin in β -catenin −/− ESCs was confirmed by western blot analysis. β -catenin −/− EpiSCs were generated from β -catenin fl/fl EpiSCs by transient transfection of the pCAG-Cre-IRES-Puro plasmid or from β -catenin −/− ESCs by culturing them in FGF2/activin condition [38] , [39] . β -catenin −/− EpiSCs were routinely maintained in the FGF2/activin condition. Construction of β-catenin mutant plasmids pcDNA3-human β-catenin and pcDNA3-human ΔNβ-catenin plasmids [40] (Addgene) were double-digested with Bam H1 and Not 1. Full-length and ΔNβ-catenin fragments were collected and ligated into the pCAG-IRES-hygro vector. The A295W and I296W point mutations [22] were introduced into full-length β-catenin and the ΔNβ-catenin mutant by PCR-driven overlap extension [41] using the two PCR primer pairs shown in Supplementary Table S1 . Floxed ΔNβ-catenin-ERT2 plasmid was constructed by insertion of the ΔNβ-catenin-ERT2 cassette into the pCAG-loxP-IRES-pac-STOP-loxP-EGFP-pA vector [42] . Full-length β-catenin or β-catenin mutants were transfected into mouse ESCs, mouse EpiSCs and human ESCs by electroporation. Drug-resistant colonies were picked and expanded to establish stable cell lines. Construction of Axin expression plasmids and Axin shRNA Mouse Axin1 and Axin2 open reading frames were amplified by PCR from CD1 EpiSCs using KOD Hot Start DNA Polymerase (EMD). Axin1 and Axin2 open reading frames were then cloned into the PiggyBac transposon vector and verified by DNA sequencing. For RNA interference of Axin1 and Axin2 in EpiSCs, shRNA constructs designed to target 21 base-pair gene-specific regions in Axin1 and Axin2 were cloned into pLKO.1-TRC vector (Addgene). The targeted sequences were as follows: Axin1, GCCACAGAAATTTGCTGAAGA; Axin2, GGTTTGCTTGTAATGGGTTCA. For overexpression of Axin1 or Axin2 in EpiSCs, 2 μg transposon vector was co-transfected with 2 μg PiggyBac-Axin1 or PiggyBac-Axin2 into EpiSCs using Lipofectamine LTX and Plus reagent (Invitrogen) according to the manufacturer’s instructions. Twenty four hours after transfection, 1 μg ml −1 puromycin was added to the cell culture medium to select for transfected colonies. For RNAi experiments, pLKO.1-TRC-based lentiviral vectors were transfected with packaging plasmids pMD2.G and psPAX2 into 293FT cells (Invitrogen) using Lipofectamine LTX and Plus reagent. Virus-containing supernatant was collected 48 h after transfection. EpiSCs were incubated in the virus supernatant supplemented with 8 μg ml −1 polybrene (Sigma) for 24 h. Supernatant was then replaced with fresh CHIR/IWR-1 medium supplemented with 1 μg ml −1 puromycin to select for transfected cells. qRT–PCR Total RNA was extracted with the RNeasy Mini Kit (Qiagen). cDNA was synthesized with 1 ng of total RNA, using the QuantiTech Rev. Transcription Kit (Qiagen). qRT–PCR was performed with Power SYBR Green PCR Master Mix (Applied Biosystems) according to the manufacturer’s instructions. Signals were detected with an ABI7900HT Real-Time PCR System (Applied Biosystems). The relative expression level was determined by the 2-ΔCT method and normalized against GAPDH . The primers used for qRT–PCR are shown in Supplementary Table S2 . Teratoma formation of mouse EpiSCs and human ESCs Mouse EpiSCs and human ESCs maintained in CHIR/XAV or CHIR/IWR-1 conditions were tested for their ability to form teratomas in immunodeficient SCID mice. Colonies were dissociated into small-cell clumps with CTK solution and cells were resuspended in PBS at a concentration of 1 × 10 7 cells per ml. Five hundred microliters of cell suspension was subcutaneously injected into right and left flank of 12-week-old NOD SCID mice (Charles River). Tumors were allowed to develop for 8 weeks. Teratomas were removed and fixed in 4% paraformaldehyde for 48 h, followed by paraffin embedding, sectioning and staining with hematoxylin and eosin (H&E). In vitro differentiation of mouse EpiSCs and human ESCs In vitro mouse EpiSC and human ESC differentiation was induced by formation of EBs. Mouse EpiSC- or human ESC-derived EBs were plated onto gelatin-coated dishes and cultured in GMEM/10% FBS medium. Spontaneously beating cardiomyocytes appeared after 2 weeks in culture. Neural differentiation of mouse EpiSCs and human ESCs was induced by culturing them on 0.1% gelatin-coated dishes in serum-free N2B27 medium [43] , [44] . Western blot and Co-IP Western blotting was performed according to a standard protocol. Nuclear and cytoplasmic proteins were extracted using NE-PER Nuclear protein Extraction Kit (Thermo). For Co-IP, cell extracts were prepared using Nonidet P-40 lysis buffer (50 mM Tris–HCl, pH 7.5, 150 mM NaCl, 0.5% Nonidet P-40, 1 mM EDTA, 10% glycerol, 1 mM Na 3 VO 4 , 50 mM NaF and protease inhibitors). The supernatant was collected and incubated with either anti-β-catenin or anti-Flag antibody for 2 h at 4 °C following incubation with protein A/G Plus-Agarose (Santa Cruz) for 1 h. The beads were then washed five times with lysis buffer and resuspended in SDS sample buffer. Primary antibodies used include the following: β-catenin (BD Bioscience, 1:2,000), phospho-Ser45 β-catenin (9564, Cell signalling, 1:500), Axin1 (AF3287, R&D, 1:1,000), Axin 2 (M-20, Santa Cruz, 1:200), histone H4 (2592, Cell signalling, 1:1,000), ERα (MC-20, Santa Cruz, 1:1,000), TCF3 (M-20, Santa Cruz, 1:1,000), actin (C-11, Santa Cruz, 1:1,000), Flag (F3165, Sigma, 1:2,000), α-tubulin (B-5-1-2, Invitrogen, 1:2,000). Full western blot images are shown in Supplementary Fig. S5 . Immunostaining Immunostaining was performed according to a standard protocol. Primary antibodies used include the following: Oct4 (C-10, Santa Cruz, 1:200), Sox2 (Y-17, Santa Cruz, 1:200), SSEA-1 (480, Santa Cruz, 1:200), GATA4 (G-4, Santa Cruz, 1:200), Nanog (R&D Systems, 1:200), βIII-tubulin (Invitrogen, 1:2,000), Myosin (MF-20, DSHB, 1:5), AFP (mouse monoclonal, Sigma) and αSMA (mouse monoclonal, Dako). Alexa Flour fluorescent secondary antibodies (Invitrogen) were used at a 1:2,000 dilution. Nuclei were visualized with DAPI or Hoechst. AP staining was performed with an alkaline phosphatase kit (Sigma) according to the manufacturer’s instructions. Promoter-enhancer reporter assay For quantifying relative Oct3/4 enhancer activities, pGL3-Oct4 DE and pGL3-Oct4 PE plasmids (gifts from Hans Schöler’s lab) were co-transfected with the Renilla vector, using the Amaxa Transfection Kit (Lonza). Dual Luciferase Assay (Promega) was performed the following day according to the manufacturer’s instructions. For quantifying relative β-catenin/Tcf transcriptional activity, pGL2-SuperTOP plasmid (gift from Randall Moon) was co-transfected with the Renilla vector and assayed accordingly. Bisulfite sequencing Genomic DNA was extracted with the QIAamp DNA Mini Kit (Qiagen). Approximately 500 ng DNA from each sample was treated with the EZ DNA methylation kit (ZYMO) to convert the unmethylated C’s to U’s. The promoter regions of Oct4, Stella and Vasa were amplified with primer sets ( Supplementary Table S3 ) [17] using the Expand High-fidelity PCR system (Roche), cloned into the pCR-BluntII-TOPO vector (Invitrogen) and sequenced with the T7 -promoter primer. DNA microarray analysis Total RNA was extracted with the RNeasy Mini Kit (Qiagen). RNA was amplified, labeled and hybridized to the GeneChip Mouse Gene 1.0 ST Array according to standard Affymetrix protocols. A DNA microarray was performed at the University of California, Los Angeles DNA Microarray core facility. The data analysis was performed using Partek Microarray Software. Accession codes: Microarray data reported in this paper have been deposited in the Gene Expression Omnibus database with the accession number of GSE31461 . How to cite this article: Kim, H. et al. Modulation of β-catenin function maintains mouse epiblast stem cell and human embryonic stem cell self-renewal. Nat. Commun. 4:2403 doi: 10.1038/ncomms3403 (2013).